Distinct Nav1.7-dependent pain sensations require different sets of sensory and sympathetic neurons Human acute and inflammatory pain requires the expression of voltage-gated sodium channel Nav1.7 but its significance for neuropathic pain is unknown. Here we show that Nav1.7 expression in different sets of mouse sensory and sympathetic neurons underlies distinct types of pain sensation. Ablating Nav1.7 gene ( SCN9A ) expression in all sensory neurons using Advillin-Cre abolishes mechanical pain, inflammatory pain and reflex withdrawal responses to heat. In contrast, heat-evoked pain is retained when SCN9A is deleted only in Nav1.8-positive nociceptors. Surprisingly, responses to the hotplate test, as well as neuropathic pain, are unaffected when SCN9A is deleted in all sensory neurons. However, deleting SCN9A in both sensory and sympathetic neurons abolishes these pain sensations and recapitulates the pain-free phenotype seen in humans with SCN9A loss-of-function mutations. These observations demonstrate an important role for Nav1.7 in sympathetic neurons in neuropathic pain, and provide possible insights into the mechanisms that underlie gain-of-function Nav1.7-dependent pain conditions. Voltage-gated sodium channels are crucial determinants of neuronal excitability and signalling. Voltage-gated sodium channels Nav1.7, 1.8 and 1.9 are expressed in peripheral neurons and have been linked to pain pathways [1] . The biophysical characteristics of Nav1.7 suggest a role in initiating action potentials in response to depolarization of sensory neurons by noxious stimuli [2] , [3] . Nav1.8 is a major contributor to the upstroke of action potentials in sensory neurons and is essential for cold pain perception [4] . Nav1.9 influences inflammatory pain thresholds by producing a persistent current that helps determine the resting membrane potential [5] . Rare human genetic conditions involving Nav1.7 mutations demonstrate its important role in pain pathways. Dominant gain-of-function mutations can cause primary erythromelalgia, resulting in burning pain and flushing [6] . Mutations associated with the condition, for example F1449V [7] and L858H [8] , result in lower thresholds for action potential firing and higher-frequency firing in sensory neurons. Other gain-of-function Nav1.7 mutations that cause defective fast inactivation may cause burning pain associated with paroxysmal extreme pain disorder (PEPD), in which mechanical stimulation triggers pain [9] . Loss-of-function recessive mutations cause congenital insensitivity to pain (CIP) and anosmia; individuals with this syndrome are of normal intelligence and can function effectively [3] , [10] . These observations highlight Nav1.7 as a potentially useful target for the development of novel analgesics. Early studies on Nav1.7 function in transgenic mice focused on the role of this channel in Nav1.8-positive nociceptors [11] . Deletion of the SCN9A gene in these neurons results in a loss of sensitivity to high-threshold noxious mechanical stimuli and major deficits in inflammatory pain. Unlike humans with global loss-of-function mutations, however, there is no deficit in noxious thermosensation. Here we have used Cre recombinase expressed in different sets of sensory and sympathetic neurons to explore modality-specific pain sensations that are dependent on the expression of Nav1.7. Advillin is an actin-binding protein that is selectively expressed within all trigeminal and dorsal root ganglion (DRG) neurons [12] , [13] . We used Cre driven by the Advillin promoter to delete Nav1.7 in all sensory neurons [14] , and compared phenotypes with mice in which Nav1.7 is deleted using Cre driven by Nav1.8 in a subpopulation of sensory neurons ( Nav1.7 Nav1.8 ) [11] . Wnt1 is expressed in neural crest cells that are the precursors of sensory and autonomic neurons [15] . This has allowed us to exploit a Wnt1-Cre mouse [16] to examine the contribution of Nav1.7 to pain behaviour in both the sensory and sympathetic neurons, where it is selectively expressed [17] . We have thus been able to define the pain modalities associated with different sets of peripheral neurons that express Nav1.7. We provide evidence that Nav1.7 may be involved at both the central as well as the peripheral terminals of sensory neurons in pain signalling. We also demonstrate an interaction between sympathetic and primary sensory neurons in acute heat sensing as well as neuropathic pain, which are both dependent upon Nav1.7 activity. These experiments provide a comprehensive mouse model of human CIP for mechanistic studies and reinforce the significance of Nav1.7 as an analgesic drug target. Pan-DRG neuron gene ablation with an Advillin-Cre mouse The expression pattern of functional Cre was first examined by crossing an Advillin-Cre knock-in-positive mouse line [14] with Rosa26 floxed-stop β-galactosidase-expressing reporter mice [18] . X-gal staining of E14.5 Advillin-Cre-positive reporter ( Advillin-Cre +/− ) mice embryos showed that Cre expression is confined to the DRG and trigeminal neurons ( Fig. 1a,b ), while no staining is seen in Advillin-Cre-negative reporter mice. Positive X-gal staining was seen in all DRG cells in sections taken from 6-week-old- Advillin-Cre +/− reporter mice ( Fig. 1c ). No positive staining was seen in other tissues sampled, including the superior cervical ganglia (SCG— Fig. 1d ). This X-gal staining seen in Advillin-Cre +/− reporter mice corroborates previous studies of expression patterns using in situ hybridization and human placental alkaline phosphatase reporter mice [12] . The expression pattern of Wnt1-Cre has been reported [16] , and was confirmed by crossing Wnt1-Cre -positive mice with Rosa26 floxed-stop β-galactosidase reporter mice. Positive X-gal staining was seen in both DRG and SCG isolated from Wnt1-Cre -positive reporter mice ( Fig. 1e,f ). A count of cells with positive staining for antibodies to neurofilament N200 protein (a marker of A-fibre-associated sensory neurons— Supplementary Fig. S1a,b ) as well as peripherin (a marker of nociceptive sensory neurons— Supplementary Fig. S1a,b ) shows no neuronal loss in Advillin-Cre +/− mice ( Supplementary Fig. S1c ). 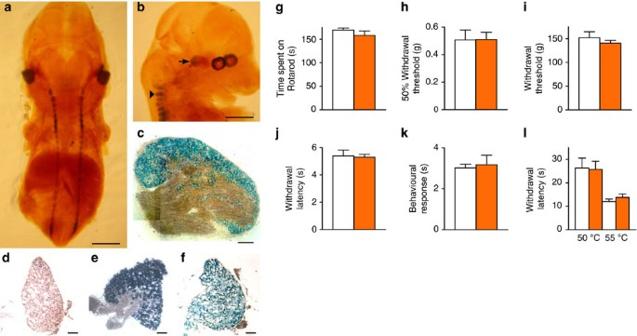Figure 1: Advillin and Wnt1 Cre expression pattern and pain behaviour of Advillin-Cre mice. (a,b) Expression pattern of Cre activity. Arrow: trigeminal, arrowhead: DRG (scale bar 1 mm). X-gal staining of Advillin-Cre positive (c) DRG and (d) SCG sections, and Wnt1-Cre positive (e) DRG and (f) SCG sections (scale bar 100 μm). Acute nociceptive responses of heterozygous Advillin-Cre (orange columns) and littermate (white columns) mice (N shown as littermate/AdCre+/−). (g) Motor coordination: Rotarod test (N=15/16). (h) Light touch: von Frey (N=15/16). (i) Mechanical pain: Randall–Selitto test (N=13/16). (j) Thermal spinal reflex: Hargreaves' test (N=15/16). (k) Noxious cooling: acetone test (N=10/11). (l) Supraspinal thermal: hotplate test at 50 and 55 °C (N=6/6). All behavioural data analysed byt-test. Results are presented as mean±s.e.m. Figure 1: Advillin and Wnt1 Cre expression pattern and pain behaviour of Advillin-Cre mice. ( a , b ) Expression pattern of Cre activity. Arrow: trigeminal, arrowhead: DRG (scale bar 1 mm). X-gal staining of Advillin-Cre positive ( c ) DRG and ( d ) SCG sections, and Wnt1-Cre positive ( e ) DRG and ( f ) SCG sections (scale bar 100 μm). Acute nociceptive responses of heterozygous Advillin-Cre (orange columns) and littermate (white columns) mice (N shown as littermate/AdCre +/− ). ( g ) Motor coordination: Rotarod test ( N =15/16). ( h ) Light touch: von Frey ( N =15/16). ( i ) Mechanical pain: Randall–Selitto test ( N =13/16). ( j ) Thermal spinal reflex: Hargreaves' test ( N =15/16). ( k ) Noxious cooling: acetone test ( N =10/11). ( l ) Supraspinal thermal: hotplate test at 50 and 55 °C ( N =6/6). All behavioural data analysed by t -test. Results are presented as mean±s.e.m. Full size image Having established that Advillin-Cre was effective in deleting genes in all sensory neurons, we examined the behaviour of the Advillin-Cre mouse line. Motor function was assessed using the Rotarod test [19] , which showed that the responses of Advillin-Cre +/− mice are the same as those of wild-type littermate controls ( Fig. 1g ). Mechanosensation assessed using von Frey filaments applied to the hindpaw and the Randall–Selitto test applied to the tail also showed normal responses in Advillin-Cre +/− mice ( Fig. 1h,i ). Finally, pain behaviour in response to noxious thermal stimuli applied to the hindpaw(s) was also normal ( Fig. 1j–l ). Behavioural responses to both short- and long-term inflammatory pain models were also normal in Advillin-Cre +/− mice ( Fig. 2a–e ). Similarly, mechanical sensitivity developed normally in response to surgically induced neuropathic pain ( Fig. 2f ). The same acute pain tests as described above were performed on Wnt1-Cre -expressing mice, which showed responses similar to wild-type littermate controls ( Supplementary Fig. S2a–f ). Wnt1-Cre mice have previously been shown to have normal behavioural responses in both inflammatory and neuropathic pain models [20] . Thus, there are no background problems in interpreting behavioural phenotypes when using these mice for gene deletion studies. 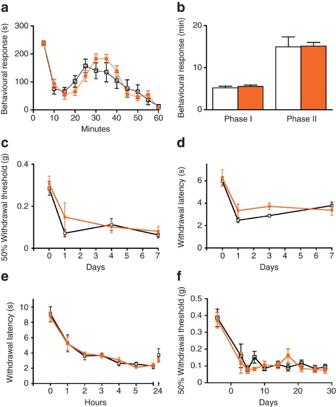Figure 2: Advillin-Cre does not affect inflammatory or neuropathic pain behaviour. Advillin-Cre+/−(orange boxes/columns), littermates (white boxes/columns). (a,b) Behavioural responses of Advillin-Cre+/−(N=12) wild-type littermate (N=8) mice following intraplantar injection of 20 μl of 5% formalin. (c) von Frey 50% threshold response of Advillin-Cre+/−(N=9) and wild-type littermate (N=8) mice following intraplantar injection of 20 μl of complete Freund's adjuvant. (d) Hargreaves' test responses of Advillin-Cre+/−mice (N=9) and wild-type littermate (N=8) mice following intraplantar injection of 20 μl of complete Freund's adjuvant. (e) Hargreaves' test response of Advillin-Cre+/−mice (N=12) and wild-type littermates (N=10) mice following intraplantar injection of 20 μl of carrageenan. (f) von Frey 50% threshold response of Advillin-Cre+/−mice (N=12) and wild-type littermates (N=10) mice following L5 SNT. All data analysed by two-way analysis of variance followed by the Bonferronipost hoctest. Results are presented as mean±s.e.m. Figure 2: Advillin-Cre does not affect inflammatory or neuropathic pain behaviour. Advillin-Cre +/− (orange boxes/columns), littermates (white boxes/columns). ( a , b ) Behavioural responses of Advillin-Cre +/− ( N =12) wild-type littermate ( N =8) mice following intraplantar injection of 20 μl of 5% formalin. ( c ) von Frey 50% threshold response of Advillin-Cre +/− ( N =9) and wild-type littermate ( N =8) mice following intraplantar injection of 20 μl of complete Freund's adjuvant. ( d ) Hargreaves' test responses of Advillin-Cre +/− mice ( N =9) and wild-type littermate ( N =8) mice following intraplantar injection of 20 μl of complete Freund's adjuvant. ( e ) Hargreaves' test response of Advillin-Cre +/− mice ( N =12) and wild-type littermates ( N =10) mice following intraplantar injection of 20 μl of carrageenan. ( f ) von Frey 50% threshold response of Advillin-Cre +/− mice ( N =12) and wild-type littermates ( N =10) mice following L5 SNT. All data analysed by two-way analysis of variance followed by the Bonferroni post hoc test. Results are presented as mean±s.e.m. Full size image Polymerase chain reaction (PCR) analysis showed that SCN9A exons 14 and 15 are deleted in cDNA isolated from DRG in homozygous floxed SCN9A , Advillin-Cre +/− mice ( Nav1.7 Advill ) but not in the littermate homozygous floxed SCN9A Advillin-Cre-negative mice ( Supplementary Fig. S3a ). However, exons 14 and 15 remain intact in the SCG that contain the cell bodies of sympathetic neurons in Nav1.7 Advill mice ( Supplementary Fig. S3b ). In contrast, exons 14 and 15 are deleted in cDNA isolated from both DRG and SCG ( Supplementary Fig. S3c,d ) in the homozygous floxed SCN9A , Wnt1-Cre -positive mice ( Nav1.7 Wnt1 ). Nav1.7 knockout mice define pain modality-specific neurons By comparing the pain behaviour of different mouse lines, it was possible to examine the role of Nav1.7 expressed in Nav1.8-positive sensory neurons ( Nav1.7 Nav1.8 ), all sensory neurons ( Nav1.7 Advill ) or sensory and sympathetic neurons ( Nav1.7 Wnt1 ). Analysis of the behavioural responses of Nav1.7 Nav1.8 Nav1.7 Advill and Nav1.7 Wnt1 mice in a number of different pain models showed that their pain phenotypes differ. Fig. 3a shows that all three Nav1.7 knockout mouse strains show pronounced analgesia in terms of noxious mechanosensation measured with a Randall–Selitto apparatus, when compared with their littermate controls. This confirms the findings of Nassar et al . [11] , who examined the Nav1.7 Nav1.8 mouse. The Randall–Selitto test results suggest that deleting Nav1.7 within Nav1.8-positive DRG neurons is sufficient to abolish responses to mechanical pain. However, the results of the acetone (noxious cooling) test ( Fig. 3b ) and Hargreaves' (thermal: spinal withdrawal reflex) test ( Fig. 3c ) show deficits in the Nav1.7 Advill and Nav1.7 Wnt1 mice, while the behavioural response of Nav1.7 Nav1.8 was not significantly different from littermate controls (confirmed by separate behavioural tests— Supplementary Fig. S4a,b ). Thus, noxious cooling-evoked behaviour and spinal withdrawal reflexes to noxious heat require Nav1.7 expression in Nav1.8-negative sensory neurons. However, this is not true for supraspinal responses to the hotplate test ( Fig. 3d —discussed below). Other work supports the view that Nav1.7 expressed within Nav1.8-positive DRG neurons contributes little to thermal nociceptive processing. Abrahamsen et al . [21] showed that behavioural responses to noxious thermal stimuli (with the exception of extreme cold) remain intact in mice in which all Nav1.8-positive neurons have been ablated with diphtheria toxin ( Nav1.8 DTA ). Additionally, in vivo electrophysiological recordings from spinal lamina V wide dynamic range (WDR) neurons in Nav1.7 Advill Nav1.7 Nav1.8 and Nav1.8 DTA mice corroborate the behavioural data. Critically, WDR responses in Nav1.7 Advill mice show that both noxious heat and mechanical stimuli are attenuated ( Fig. 3e,f ). In contrast, only mechanically evoked and not heat-evoked WDR responses are attenuated in both Nav1.7 Nav1.8 mice [11] and Nav1.8 DTA mice [21] . This demonstrates clearly that Nav1.7 expressed in Nav1.8-positive DRG neurons is essential for processing noxious mechanical stimuli while Nav1.7 in Nav1.8-negative DRG neurons is essential for processing noxious thermal stimuli. 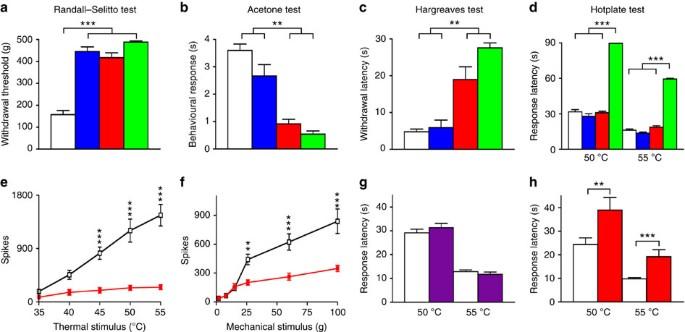Figure 3: Nociceptive responses of different tissue-specific Nav17 KO mice. Littermate (white columns), Nav1.7Nav1.8(blue columns), Nav1.7Advill(red columns) and Nav1.7Wnt1(green columns), N shown as littermate/Nav1.7Nav1.8/Nav1.7Advill/Nav1.7Wnt1. (a) Randall–Selitto test (noxious mechanical stimulus;N=23/6/13/5). (b) Acetone cooling test (noxious cooling stimulus;N=29/6/7/5). (c) Hargreaves' test (spinal noxious heat stimulus;N=22/6/7/7). (d) Hotplate test (supraspinal noxious heat stimulus;N=37/8/19/10):in vivoelectrophysiological spinal cord recording from Nav1.7Advill(red boxes) and littermate (white boxes) mice. (e) Thermally evoked WDR responses (N=6 per group). (f) Mechanically evoked WDR responses (N=6 per group). (g) Hotplate test following 6-OHDA treated (purple column,N=10) and untreated (white column,N=12) C57/Black6 mice. (h) Hotplate test of Nav1.7Advill(red column,N=7) and littermate mice (white column,N=12) following chemical 6-OHDA treatment. (a–d) Data analysed byt-test, (e–h) data analysed by two-way analysis of variance followed by the Bonferronipost hoctest. Results are presented as mean±s.e.m. ***P<0.01 and ***P<0.001 (individual points). Figure 3: Nociceptive responses of different tissue-specific Nav17 KO mice. Littermate (white columns), Nav1.7 Nav1.8 (blue columns), Nav1.7 Advill (red columns) and Nav1.7 Wnt1 (green columns), N shown as littermate/Nav1.7 Nav1.8 /Nav1.7 Advill /Nav1.7 Wnt1 . ( a ) Randall–Selitto test (noxious mechanical stimulus; N =23/6/13/5). ( b ) Acetone cooling test (noxious cooling stimulus; N =29/6/7/5). ( c ) Hargreaves' test (spinal noxious heat stimulus; N =22/6/7/7). ( d ) Hotplate test (supraspinal noxious heat stimulus; N =37/8/19/10): in vivo electrophysiological spinal cord recording from Nav1.7 Advill (red boxes) and littermate (white boxes) mice. ( e ) Thermally evoked WDR responses ( N =6 per group). ( f ) Mechanically evoked WDR responses ( N =6 per group). ( g ) Hotplate test following 6-OHDA treated (purple column, N =10) and untreated (white column, N =12) C57/Black6 mice. ( h ) Hotplate test of Nav1.7 Advill (red column, N =7) and littermate mice (white column, N =12) following chemical 6-OHDA treatment. ( a–d ) Data analysed by t -test, ( e–h ) data analysed by two-way analysis of variance followed by the Bonferroni post hoc test. Results are presented as mean±s.e.m. *** P <0.01 and *** P <0.001 (individual points). Full size image Nav1.7 is expressed in sympathetic as well as sensory neurons [2] , [17] . By using the Wnt1 promoter to drive Cre expression it is possible to delete genes in neural crest derivatives including autonomic and sensory neurons. Therefore, we could identify any role for Nav1.7 in sympathetic neurons by comparing the phenotype of Nav1.7 Advill and Nav1.7 Wnt1 mice. Interestingly, only Nav1.7 Wnt1 mice have an attenuated response to the hotplate test ( Fig. 3d ), which is a measure of supra-spinal responses [22] to damaging thermal stimuli rather than a spinal reflex involving only cells in the spinal cord [23] . In contrast, Nav1.7 Advill (as well as Nav1.7 Nav1.8 ) mice show normal hotplate pain behaviour ( Fig. 3d ). However, this does not mean that Nav1.7 in sympathetic neurons alone confers sensitivity to the hotplate test. Chemical sympathectomy using 6-hydroxydopamine (6-OHDA) [24] in wild-type mice has no effect on behavioural responses to the hotplate test ( Fig. 3g ) or any other acute pain thresholds tested ( Supplementary Fig. S5a–f ). However, when chemical sympathectomy is combined with the deletion of sensory neuron Nav1.7 in Nav1.7 Advill mice, the hotplate response is diminished ( Fig. 3h ). Thus, only when Nav1.7 expression is lost in both sensory and sympathetic neurons do mice become unresponsive ( Fig. 3d ). Despite the role of the sympathetic nervous system in thermoregulation, the core temperature and skin temperature of Nav1.7 Wnt1 ( Fig. 4a ) and 6-OHDA-treated mice ( Supplementary Fig. S5g ) were found to be normal. 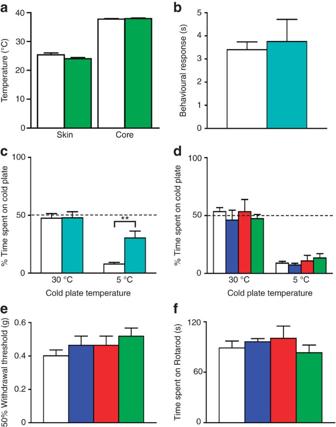Figure 4: Behavioural responses of different tissue-specific Nav1.7 and Nav1.8 KO mice to cooling and extreme cold. N shown as littermate/Nav1.7Wnt1. (a) Nav1.7Wnt1(green columns) and littermate (white columns) core (N=12/13) and skin temperature (N=12/9). (b) Behavioural response of Nav1.8 KO (turquoise column,N=5) and littermate (white column,N=7) mice to the acetone cooling test. (c) Behavioural response of Nav1.8 KO (turquoise columns,N=8) and littermate (white columns,N=6) thermal place preference test. (d–f) Littermate (white columns), Nav1.7Nav1.8(blue columns), Nav1.7Advill(red columns), Nav1.7Wnt1(green columns) N shown as littermate/Nav1.7Nav1.8/Nav1.7Advill/Nav1.7Wnt1. (d) Behavioural response of all three Nav1.7 tissue-specific knockout mice to thermal place preference test (N=15/8/8/8). (e) Behavioural response of all three Nav1.7 tissue-specific knockout mice to the von Frey test. (f) Behavioural response of all three Nav1.7 tissue-specific knockout mice to the Rotarod test (N=23/8/13/9). (a,b) Data analysed byt-test, (c–f) data analysed by two-way analysis of variance followed by the Bonferronipost hoctest. Results are presented as mean±s.e.m. **P<0.01 (individual points). Figure 4: Behavioural responses of different tissue-specific Nav1.7 and Nav1.8 KO mice to cooling and extreme cold. N shown as littermate/Nav1.7 Wnt1 . ( a ) Nav1.7 Wnt1 (green columns) and littermate (white columns) core ( N =12/13) and skin temperature ( N =12/9). ( b ) Behavioural response of Nav1.8 KO (turquoise column, N =5) and littermate (white column, N =7) mice to the acetone cooling test. ( c ) Behavioural response of Nav1.8 KO (turquoise columns, N =8) and littermate (white columns, N =6) thermal place preference test. ( d–f ) Littermate (white columns), Nav1.7 Nav1.8 (blue columns), Nav1.7 Advill (red columns), Nav1.7 Wnt1 (green columns) N shown as littermate/Nav1.7 Nav1.8 /Nav1.7 Advill /Nav1.7 Wnt1 . ( d ) Behavioural response of all three Nav1.7 tissue-specific knockout mice to thermal place preference test ( N =15/8/8/8). ( e ) Behavioural response of all three Nav1.7 tissue-specific knockout mice to the von Frey test. ( f ) Behavioural response of all three Nav1.7 tissue-specific knockout mice to the Rotarod test ( N =23/8/13/9). ( a , b ) Data analysed by t -test, ( c–f ) data analysed by two-way analysis of variance followed by the Bonferroni post hoc test. Results are presented as mean±s.e.m. ** P <0.01 (individual points). Full size image We next examined the responses of the three Nav1.7 knockout lines to noxious cold stimuli, and compared them with a global Nav1.8 knockout mouse that is known to lose sensitivity to noxious cold [4] . Interestingly, the Nav1.8 knockout mouse responded to acetone-induced cooling in the same way as littermate control mice ( Fig. 4b ), but showed an attenuated response to extreme cold ( Fig. 4c ). In contrast, all three Nav1.7 conditional knockout mouse lines that showed attenuated responses to acetone-induced cooling ( Fig. 3b ) avoided extreme cold like their littermate controls ( Fig. 4d ). Thus, noxious cold sensation is not Nav1.7 dependent. Finally, all three Nav1.7 knockout mouse lines showed normal responses to light touch and motor coordination ( Fig. 4e,f ), reinforcing the link between Nav1.7 and pain rather than innocuous somatosensation. Substance P release from DRG neurons is Nav1.7 dependent The functional consequences of deleting Nav1.7 in DRG neurons were further examined electrophysiologically. Nav1.7 Advill DRG neurons showed a significant average reduction in tetrodotoxin (TTX)-sensitive sodium current amplitude, whereas TTX-resistant sodium currents were unchanged ( Fig. 5a ). Complete current–voltage relationships are shown in Fig. 5b,c . Approximately 30% of small DRG neurons have been shown to be electrically silenced by the deletion of Nav1.7 in Nav1.8-positive DRG neurons [25] . We found that electrically stimulated polysynaptic peripheral input into spinal lamina V WDR neurons no longer resulted in wind-up ( Fig. 5d )—an N -methyl- D -aspartate receptor-mediated form of long-term sensitization that requires substance P release from sensory neurons [26] . Substance P release from sensory neurons was therefore measured in Nav1.7 Advill mice. Strikingly, electrical stimulation of isolated sciatic nerve roots failed to induce increased substance P release into the dorsal horn of Nav1.7 Advill mice ( Fig. 5e ). 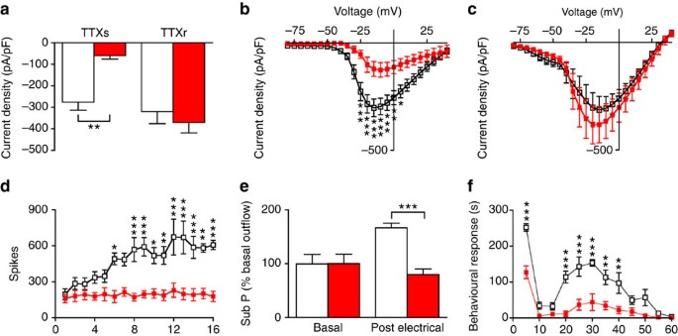Figure 5: Reduced electrically evoked wind-up and substance P release in the spinal cord of Nav1.7Advillmice. Littermate (white columns/boxes), Nav1.7Advill(red columns/boxes) N shown as littermate/Nav1.7Advill. (a) TTX-sensitive and TTX-resistant inward sodium currents recorded from Nav1.7AdvillDRG neurons (N=11/6) Current–voltage relationships for sodium currents in littermate control (N=11) and Nav1.7AdvillDRG neurons (N=6) in the presence (b) or absence (c) of 500 nM TTX. (d) WDR spinal recording from Nav1.7Advilland littermate mice in response to electrical stimulation of the sciatic nerve (N=6 per group). (e) Electrically evoked substance P release into the dorsal horn measured by radioimmunoassay in Nav1.7Advilland littermate mice (N=7/8). (f) First and second phase responses observed in Nav1.7Advillmice after intraplantar injection of 20 μl of 5% formalin (N=6/5). All data analysed by two-way analysis of variance followed by the Bonferronipost hoctest. Results are presented as mean±s.e.m. *P<0.05, **P<0.01 and ***P<0.001 (individual points). Figure 5: Reduced electrically evoked wind-up and substance P release in the spinal cord of Nav1.7 Advill mice. Littermate (white columns/boxes), Nav1.7 Advill (red columns/boxes) N shown as littermate/Nav1.7 Advill . ( a ) TTX-sensitive and TTX-resistant inward sodium currents recorded from Nav1.7 Advill DRG neurons ( N =11/6) Current–voltage relationships for sodium currents in littermate control ( N =11) and Nav1.7 Advill DRG neurons ( N =6) in the presence ( b ) or absence ( c ) of 500 nM TTX. ( d ) WDR spinal recording from Nav1.7 Advill and littermate mice in response to electrical stimulation of the sciatic nerve ( N =6 per group). ( e ) Electrically evoked substance P release into the dorsal horn measured by radioimmunoassay in Nav1.7 Advill and littermate mice ( N =7/8). ( f ) First and second phase responses observed in Nav1.7 Advill mice after intraplantar injection of 20 μl of 5% formalin ( N =6/5). All data analysed by two-way analysis of variance followed by the Bonferroni post hoc test. Results are presented as mean±s.e.m. * P <0.05, ** P <0.01 and *** P <0.001 (individual points). Full size image The deficits in sensory neuron function and lack of wind-up may be related to pain behaviour assessed using the formalin test. This comprises a first phase of paw licking driven by nociceptor activation followed by a second phase associated with spinal cord hypersensitivity mediated by chemical messengers including substance P [27] . Nav1.7 Advill mice show a striking ~75% decrease in behavioural responses during phase II of the formalin test ( Fig. 5f ), which is similar to the phase II phenotype of both Nav1.7 Nav1.8 and Nav1.8 DTA mice [11] , [21] . Interestingly, Nav1.7 Advill mice show a large phase I behavioural deficit (~50% decrease in behavioural responses) whereas Nav1.7 Nav1.8 mice [11] and Nav1.8 DTA mice [21] do not. This suggests an important role for Nav1.7 expressed in Nav1.8-negative DRG neurons during the initial nociceptive phase of the formalin test [26] . Neuropathic pain requires Nav1.7 in sympathetic neurons Previously Nassar et al . [11] showed that Nav1.7 Nav1.8 mice develop neuropathic pain normally. Thus, Nav1.7 expressed in Nav1.8-positive neurons, while making a major contribution to inflammatory pain, does not contribute to neuropathic pain [11] . Importantly, Nav1.8 DTA mice also develop neuropathic pain normally, showing that Nav1.8-positive neurons are not required for the development of neuropathic pain [28] . However, recently a blocker of inactivated Nav1.7 has been claimed to reverse mechanical hyperalgesia associated with neuropathic pain models [28] . This suggests a possible contribution to neuropathic pain of Nav1.7 expressed in Nav1.8-negative DRG neurons, which remain intact within Nav1.7 Nav1.8 mice. Therefore, Nav1.7 Advill mice in which Nav1.7 is lost in all sensory neurons were examined. Nav1.7 Advill mice developed mechanical hypersensitivity to the same extent as normal littermates, following spinal nerve transection (SNT) at the fifth lumbar segment—a model of neuropathic pain [29] , [30] , [31] ( Fig. 6a ). Thus, Nav1.7 in sensory neurons is not required for the development of neuropathic pain. In contrast, Nav1.7 Wnt1 mice show a pronounced attenuation in the development of mechanical sensitization and return to baseline behaviour (±10%) within 10 days following surgery ( Fig. 6b ). This set of observations demonstrate that Nav1.7 expression in sympathetic neurons is essential for the establishment of neuropathic pain. An important role for sympathetic neurons in neuropathic pain is further demonstrated by the ability of a chemical sympathectomy to partially alleviate mechanical hypersensitivity in Nav1.7 Wnt1 littermate mice following SNT ( Fig. 6c ). In these experiments, neuropathic pain was established for 28 days, followed by chemical sympathectomy. A substantial, if incomplete, reversal of mechanical hypersensitivity was observed consistent with a sympathetic sensory interaction contribution to the establishment of neuropathic pain. These results may help explain the apparent utility of Nav1.7 antagonists in treating neuropathic pain [27] . 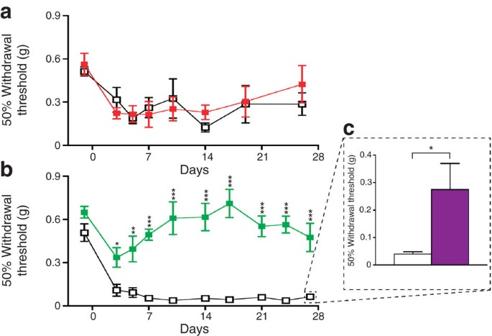Figure 6: Behavioural responses of Nav1.7Advilland Nav1.7Wnt1mice following L5 SNT. (a) Mechanical sensitization following L5 SNT of Nav1.7Advill(red boxes,N=6) and littermate (white boxes,N=9) mice. (b) Mechanical sensitization following L5 SNT of Nav1.7Wnt1(green boxes,N=9) and littermate (white boxes,N=12) mice. (c) Mechanical sensitization in littermate mice treated with 6-OHDA (purple column,N=6) or vehicle (white column,N=6) 28 days after L5 SNT surgery. All analysed by two-way analysis of variance followed by the Bonferronipost hoctest. Results are presented as mean±s.e.m. *P<0.05, **P<0.01 and ***P<0.001 (individual points). Figure 6: Behavioural responses of Nav1.7 Advill and Nav1.7 Wnt1 mice following L5 SNT. ( a ) Mechanical sensitization following L5 SNT of Nav1.7 Advill (red boxes, N =6) and littermate (white boxes, N =9) mice. ( b ) Mechanical sensitization following L5 SNT of Nav1.7 Wnt1 (green boxes, N =9) and littermate (white boxes, N =12) mice. ( c ) Mechanical sensitization in littermate mice treated with 6-OHDA (purple column, N =6) or vehicle (white column, N =6) 28 days after L5 SNT surgery. All analysed by two-way analysis of variance followed by the Bonferroni post hoc test. Results are presented as mean±s.e.m. * P <0.05, ** P <0.01 and *** P <0.001 (individual points). Full size image The apparently normal phenotype of humans with SCN9A loss-of-function mutations, apart from anosmia and loss of pain sensation, has focused attention on Nav1.7 as a plausible analgesic drug target. Ablation of the channel using the Cre-loxP system in mice leads to silencing of a significant set of sensory neurons [25] . We found that TTX-sensitive current densities were reduced in sensory neurons that no longer express Nav1.7. More surprisingly, we found that substance P release into the dorsal horn of the spinal cord evoked by electrical stimulation was completely abolished in the absence of Nav1.7, leading to a loss of wind-up and centrally mediated pain sensitization. In the olfactory system, Weiss et al . [10] have shown that while olfactory neurons support action potential propagation in the absence of Nav1.7, the release of neurotransmitter from olfactory neurons is completely abolished, leading to anosmia. A similar deficit may occur in DRG sensory neurons. Thus, Nav1.7 may contribute to pain signalling by DRG neurons in three ways: (1) by recruiting Nav1.8 to transmit noxious input into the spinal cord [1] , [2] ; (2) by supporting action potential propagation [25] , [32] and (3) by regulating neurotransmitter release at central terminals [10] . In terms of responses to innocuous stimuli and motor function, the ablation of Nav1.7 in all sensory and sympathetic neurons is without effect ( Fig. 4e,f ). However, threshold withdrawal behavioural responses to noxious pressure require Nav1.7 in a set of sensory neurons that express Nav1.8. This corroborates previous findings in Nav1.7 Nav1.8 mice [11] and Nav1.8 DTA mice [21] . Reflex threshold withdrawal responses to noxious heat are dependent on Nav1.7 expression in a different set of sensory neurons that do not express Nav1.8, an observation consistent with cell ablation studies [21] . Noxious cold is the sole pain modality that is Nav1.7 independent ( Fig. 4d ), confirming a previously described role for Nav1.8, which is sensitized at low temperatures [4] ( Fig. 4c ). Responses to noxious cooling associated with the application of acetone, however, are not dependent on Nav1.8 ( Fig. 4b ), but depend upon Nav1.7 expression in Nav1.8-negative sensory neurons. Acute pain has a clear survival function. Inflammatory pain has a positive role in enhancing self-protection and wound healing, but may cause considerable suffering in chronic inflammatory conditions such as arthritis. It has been established that Nav1.7 expressed in Nav1.8-positive neurons has an essential role in inflammatory pain. Interestingly, thermal hyperalgesia, but not threshold noxious heat sensing, is mediated by Nav1.7 in the Nav1.8-positive population. This observation confirms that distinct cells and wiring patterns are associated with acute and sensitized thermosensation [21] . 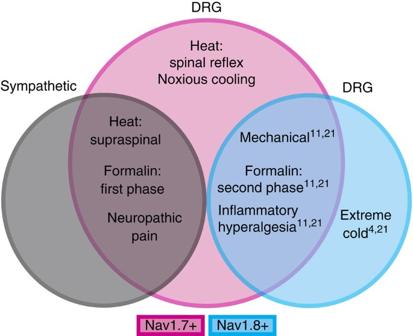Figure 7: The neuron-specific role of Nav1.7 in different pain states. Nav1.7 expressed in Nav1.8-positive sensory neurons (blue) is required for mechanical pain as well as inflammatory thermal and mechanical hyperalgesia11,21. Nav1.7 expressed in Nav1.8-negative neurons (red) is required for thermal acute pain sensing (but not extreme cold, which is dependent on Nav1.84,21). A contribution of both sensory and sympathetic (grey) Nav1.7-mediated signalling is required for neuropathic pain and responses to the hotplate test. Figure 7 summarizes the relationship between different types of pain sensation and the expression patterns of sodium channels Nav1.7 and Nav1.8. Figure 7: The neuron-specific role of Nav1.7 in different pain states. Nav1.7 expressed in Nav1.8-positive sensory neurons (blue) is required for mechanical pain as well as inflammatory thermal and mechanical hyperalgesia [11] , [21] . Nav1.7 expressed in Nav1.8-negative neurons (red) is required for thermal acute pain sensing (but not extreme cold, which is dependent on Nav1.8 [4] , [21] ). A contribution of both sensory and sympathetic (grey) Nav1.7-mediated signalling is required for neuropathic pain and responses to the hotplate test. Full size image One of the least understood and most problematic aspects of pain remains neuropathic pain. This may be because a variety of different mechanisms sensitize pain pathways after nerve damage. Nav1.7 expressed in Nav1.8-positive nociceptors is not required for the development of neuropathic pain in mouse models [11] , and the studies reported here show that Nav1.7 deletion in all sensory neurons also does not significantly impair the development of neuropathic pain. As the number of CIP patients is very limited, there is no information on the importance of Nav1.7 for the development of neuropathic pain in humans. We wondered if Nav1.7 in the sympathetic nervous system contributed to neuropathic pain, as early studies in rodents [33] had made a compelling case for a sympathetic contribution to this type of pain. Interestingly, ablation of Nav1.7 in both sensory and sympathetic neurons markedly diminished neuropathic pain in the SNT model investigated here [29] , [30] . This observation demonstrates an interaction between sympathetic and sensory neurons to produce neuropathic pain that is represented schematically in Fig. 7 . Interestingly, pain behaviour evoked by the hotplate test is also dependent on Nav1.7 in sympathetic and sensory neurons. Behavioural responses to the hotplate test have been shown to be supraspinally integrated [22] , [23] , [34] . A number of experimental manipulations specifically affect the hotplate behavioural response, but not reflex heat-evoked behaviour (typically tail-flick) [34] , [35] , [36] , [37] . Animals in which nerve growth factor (NGF) depletion leads to loss of sensory and sympathetic neurons also show a loss of hotplate sensitivity while mechanical thresholds and thermal reflex behaviour are unaffected [38] . NGF is not required for the survival of parasympathetic neurons [39] . This is consistent with a role for sympathetic neurons rather than other autonomic neurons in this pain behaviour. Silencing sympathetic and some sensory neurons by deleting VGLUT2 with Cre recombinase driven by the tyrosine hydroxylase promoter also causes a loss of hotplate sensitivity while acute mechanical pain remains intact [40] . In contrast, selectively deleting VGLUT2 using Nav1.8-Cre results in a behavioural phenotype where mechanical pain behaviour is lost while thermal pain remains intact [41] . These findings directly mirror the behavioural phenotypes associated with selective deletion of Nav1.7 within different neuronal subpopulations ( Fig. 7 ). The role of the sympathetic nervous system in pain pathways has been confirmed in some rat models of neuropathic pain [33] . Clinical studies have also shown a role for the sympathetic nervous system in acute human pain, for example, post-surgical pain [42] . General interest in the role of the sympathetic nervous system in pain pathways has diminished because sympathetic block has little effect in many human studies [26] . Our results suggest that a combination of sensory and sympathetic block may prove to be more effective in treating some pain states than a sensory block alone, perhaps because complete sensory block may be hard to achieve. How sympathetic and sensory neurons interact to enhance pain sensations is unclear; interactions at nerve terminals, cell bodies and centrally have all been invoked as possible mechanisms [43] . Interactions between sympathetic neurons and the neuronal somata of DRG neurons (Dogiel's arborizations) have been described in normal animals since the era of Ramón y Cajal [44] . Sprouting and specific interactions with sensory neurons by sympathetic neurons have been observed in several chronic pain models and recently quantitated with reporter mice [45] . Complex regional pain syndrome characterized by chronic burning pain and flushing in limbs supports the view that sympathetic input may contribute to pain, although the role of Nav1.7 has not been explored in this condition [26] . How do these findings relate to known human Nav1.7-dependent pain pathologies? It is striking that the principal sensation associated with all gain-of-function Nav1.7 mutations is burning pain. A possible explanation for this is that the heat-sensing subset of Nav1.7-expressing (Nav1.8 negative) sensory neurons show lower thresholds of activation than the Nav1.7-expressing Nav1.8-positive set of classical nociceptors linked to noxious mechanosensation. Interestingly, sympathetic block is effective in the treatment of some erythromelalgia cases, consistent with a contribution by sympathetic neurons to acute heat sensing (Bang et al . [46] and references therein). Overexpression studies of gain-of-function Nav1.7 erythromelalgia-associated mutant channels in SCG neuronal somata have shown diminished excitability of sympathetic neurons, although it is unclear if lower physiological levels of Nav1.7 expression also silence sympathetic neurons. [8] PEPD is also characterized by a burning pain evoked principally by mechanical stimuli. The association of PEPD with paroxysms of rectal, ocular or sub-mandibular pain with flushing could be related to the sympathetic contribution to this condition. [2] The Harlequin-like nature of flushing also implicates the autonomic nervous system (see, for example, Drummond and Lance [47] ). Age-related alterations in autonomic nervous system function could also be a factor in time of onset of primary erythromelalgia, which is remarkably variable in different patients [48] . Finally, the ability to abolish all pain modalities in mice that fail to express Nav1.7 in the periphery provide a useful model of CIP for mechanistic studies, and confirms the utility of mouse models of human disease for mechanistic studies. These data confirm the potential of Nav1.7 as an analgesic drug target not only for acute and inflammatory pain but also for neuropathic pain. Cre expression Cre expression was visualized using Rosa26 floxed-stop β-galactosidase reporter mice [18] . Tissues were removed and stained as described previously [49] . Briefly, animals were terminally anaesthetized using sodium pentobarbitone (Rhône Mérieux), before the thoracic cavity was opened, the right atrium nicked and the animal perfused, via the left ventricle, with 20 ml of ice-cold PBS followed by 20 ml of ice-cold 4% paraformaldehyde (PFA) in PBS. Organs were removed from their surrounding tissue, rinsed in PBS and fixed in ice-cold 4% PFA for 10–60 min. All tissues were stored in 30% sucrose+0.02% sodium azide at 4 °C before sectioning. Slides were washed in PBS before overnight staining with X-gal solution (5 mM potassium ferricyanide, 5 mM potassium ferrocyanide, 2 mM MgCl 2 and 0.5 mg ml −1 X-gal in dimethyl formamide in PBS) at 35 °C. Slides were washed three times in PBS before mounting. Genotyping Genomic DNA was isolated from ear or DRG. Nav1.7 was detected by PCR as described previously [11] . The primers used were the following: Advillin wild-type (480 bp) and Advillin-Cre (180 bp) fragments 1 • 5′-CCCTGTTCACTGTGAGTAGG-3′ (Advillin forward) 2 • 5′-AGTATCTGGTAGGTGCTTCCAG-3′ (Advillin wild-type reverse) 3 • 5′-GCGATCCCTGAACATGTCCATC-3′ (Advillin-Cre reverse). Wnt1-Cre fragment (629 bp) 1 • 5′-ATCCGAAAAGAAAACGTTGA-3′ (forward) 2 • 5′-ATCCAGGTTACGGATATAGT-3′ (reverse). Nav1.7 wild-type fragment (317 bp), Nav1.7 floxed fragment (461 bp) and Nav1.7 knockout fragment (395 bp) 1 • 5′-CAGAGATTTCTGCATTAGAATTTGTTC-3′ (Nav1.7 forward) 2 • 5′-AGTCTTTGTGGCACACGTTACCTC-3′ (Nav1.7 wild-type/floxed reverse) 3 • 5′-GTTCCTCTCTTTGAATGCTGGGCA-3′ (Nav1.7 knockout reverse). Behavioural experiments All tests were approved by the United Kingdom Home Office Animals (Scientific Procedures) Act 1986. Experiments were conducted using both male and female wild-type littermate and knockout mice, all of which were at least 6 weeks old when tested. Observers who performed behavioural experiments were blind to the genotype of the animals. The production of the SCN9A floxed mice has been described earlier [11] ; Nav1.8-Cre mice are described in Stirling et al . [49] ; Wnt1-Cre mice are described in Danielian et al . [16] Advillin reporter mice are described in Hasegawa et al . [12] and Advillin-Cre mice in Zhou et al . [14] Nav1.8 global knockout mice were described in Akopian et al . [50] Motor coordination, thermal and mechanical nociceptive, was assessed as described previously [11] , [51] . Briefly, animals were acclimatized to the test chambers before testing. Rotarod : Animals were placed onto the Rotarod at 4 r.p.m., which was then accelerated to a maximum of 40 r.p.m. within 90 s, with a cutoff of 120 s. Hargreaves' thermal test : The animal's hindpaw was exposed to an intense light beam and the withdrawal latency recorded. Hotplate : Animals were exposed to either a 50°C or a 55°C chamber floor and the withdrawal latency recorded. Thermal Place Preference (BioSeb, France) was used to assess cold avoidance. Von Frey : The up-down method described by Chaplan et al . [52] was used to determine a 50% response threshold. Randall–Selitto test : A blunt probe was used to apply force approximately midway along the tail. Formalin test Twenty microlitres of 5% formalin was injected into the hindpaw (intraplanter). Spontaneous nocifensive behavioural responses were recorded for 60 min post injection. Neuropathic pain model A modified version of the Kim and Chung [31] model of peripheral neuropathy was adapted for use on mice [29] , [30] . Thermal and mechanical thresholds were recorded at baseline and up to 28 days post surgery. Chemical sympathectomy 6-OHDA (Sigma) was dissolved in sterile saline containing 0.01% (w/v) ascorbic acid (vehicle) and was injected intraperitoneally at a concentration of 200 mg kg −1 (ref. 53 ). Control mice received an equivalent volume of vehicle alone. To verify the effectiveness of this treatment in depleting norepinephrine, spleens were collected and analysed for the presence of norepinephrine by mass spectrometry. Spinal cord electrophysiology In vivo electrophysiological recordings were obtained from single WDR neurons in lamina V within the L3–L5 region of the spinal cord of anaesthetized mice [54] . Neuronal activity in response to a train of 16 electrical stimuli (2 ms wide pulses at 0.5 Hz), delivered transcutaneously by means of pins inserted into the hindpaw, was recorded. Von Frey filaments and heated water jets were applied to the hindpaw for a period of 10 s to evoke mechanical and thermal nociceptive responses, respectively. The release of substance P from dorsal horn slices was measured as described previously [55] . Briefly, the lumbosacral spinal cord was excised and longitudinally hemisected, producing a horizontal slice with L4 and L5 dorsal roots attached. One slice was obtained from each animal, mounted in the central compartment of a three-compartment chamber and continuously superfused (1 ml min −1 ) with oxygenated (95% O 2 +5% CO 2 ) Krebs' solution (in mol l −1 : NaCl, 118; KCl, 4; MgSO 4 , 1.2; KH 2 PO 4 , 1.2; NaHCO 3 , 25; CaCl 2 , 2.5 and glucose, 11) containing 0.1% BSA, 20 μg ml −1 bacitracin, 100 μM captopril, 1 μM phosphoramidon and 6 μM dithiothreitol (Sigma, UK). BSA and protease inhibitors were added to minimize loss of detectable substance P through surface adhesion and to prevent degradation. The dorsal roots were then electrically stimulated (20 V, 0.5 ms, 1 Hz for 8 min). Superfusates were concentrated using C18 Sep-Pak reverse phase silica gel cartridges (Waters Associates, Watford, UK) and substance P measured by radioimmunoassay. Statistics Data were analysed using the GraphPad Prism 4. Student's t -test (two-tailed) was used for comparison of difference between two distributions. Multiple groups were compared using one-way or two-way analysis of variance with the Bonferroni post hoc test. Immunocytochemistry DRGs were excised from animals, fresh frozen in optimal cutting temperature compound (OCT), sectioned and post-fixed in 4% PFA for 5 min and then washed in PBS containing 30% sucrose. Serial 10-μm sections were mounted on sequential slides and air-dried for at least 2 h at room temperature. Slides were washed in PBS+0.3% Triton X-100, blocked in 10% goat serum in PBS+0.3% Triton for 1 h at room temperature and incubated in the primary antibody, diluted in the same blocking solution, overnight at 4 °C. After washing in PBS+0.3% Triton X-100, bound primary antibodies were detected by incubating with the secondary antibody at room temperature for 2 h. The slides were then washed in PBS+0.3% Triton X-100 and mounted using aqueous mounting solution. The following primary antibodies were used: 1 • Peripherin, immunoglobulin G (IgG) mouse monoclonal anti-peripherin (Sigma, UK, P-5117), 1:1,000 dilution. 2 • N200, IgG rabbit anti-neurofilament 200 (Sigma, UK, N4142), 1:200 dilution. The following secondary antibodies were used: 1 • Alexa594, monoclonal goat anti-rabbit IgG (Invitrogen, UK, 11037), 1:1,000 dilution. 2 • Alexa488, monoclonal goat anti-mouse IgG (Invitrogen, UK, A11017), 1:1,000 dilution. PCR analysis of mRNA Total RNA was isolated from DRG. Reverse transcription was performed with 1 μg of RNA by using the iScript Select cDNA synthesis kit (Bio-Rad, catalogue #170–8896). The Nav1.7 wild-type fragment (1007 bp) and knockout fragment (478 bp) were detected by PCR with the following primers: 1 • 5-CCATGGTGGTACAGATTTGCT-3 (forward) 2 • 5-CTTATCTCCGCAAGGGTACG-3 (reverse). Cell culture DRGs from all spinal levels were dissected from adult mice killed by CO 2 asphyxiation and prepared using a standard enzymatic dissociation procedure as described [49] . Briefly, following incubation in a Dispase (Gibco)/collagenase (type XI, Sigma) mix for 40 min the ganglia were mechanically triturated using a 1-ml Gilson pipette. The ganglia were centrifuged and resuspended in Dulbecco's modified Eagle's media supplemented with 10% fetal bovine serum, 1% Glutamax, 1% penicillin/streptomycin and 125 ng ml −1 NGF. For electrophysiological recording, dissociated neurons were plated on 35-mm plastic dishes (Nunc, Denmark) coated with poly- L -lysine and laminin and used up to 24 h after plating. For electrophysiological recording, dissociated neurons were plated on 35-mm plastic dishes (Nunc, Denmark) coated with poly- L -lysine and laminin and used up to 24 h after plating. Whole-cell recording Experiments were performed blind to genotype. The external solution contained (in mM): 35 NaCl, 105 CholineCl, 3 KCl, 1 MgCl 2 , 1 CaCl 2 , 10 glucose and 10 HEPES, pH adjusted to 7.3 and osmolarity to 320 osM l −1 with NaOH and glucose, respectively. Pipettes were filled with a solution containing (in mM): 140 CsF, 10 NaCl, 2 MgCl 2 , 0.1 CaCl 2 , 1.1 EGTA, 10 HEPES, pH adjusted to 7.2 and osmolarity to 310 osM with CsOH and glucose, respectively. Pipette resistances were 1.8–2.5 MΩ when filled with internal solution and pipette tips were coated in Sylgard to reduce capacitance. Recordings were made at room temperature (20–22 °C). Data acquisition and analysis Data were acquired and analysed using the pClamp software (version 8.0; Axon Instruments). Currents were recorded from small cells (<25 μm) using an Axopatch (200 series) patch clamp amplifier, filtered at 5 kHz and sampled at 20 kHz. The series resistance was compensated (60–75%). Cells were depolarized to a variety of potentials (−80 to +40 mV) from a holding potential of −120 mV. The TTX-sensitive sodium current was determined as the current that was sensitive to block by 500 nM TTX and was obtained by digitally subtracting the TTX-resistant component from the total inward current. The current density was obtained by dividing the peak current by the cell capacitance as read from the amplifier. Current densities were obtained by dividing the current at each potential by the cell capacitance as read from the amplifier. How to cite this article: Minett, M.S. et al . Distinct Nav1.7-dependent pain sensations require different sets of sensory and sympathetic neurons. Nat. Commun. 3:791 doi: 10.1038/ncomms1795 (2012).